Disease-associatedKIF3Avariants alter gene methylation and expression impacting skin barrier and atopic dermatitis risk Single nucleotide polymorphisms (SNPs) in the gene encoding kinesin family member 3A, KIF3A , have been associated with atopic dermatitis (AD), a chronic inflammatory skin disorder. We find that KIF3A SNP rs11740584 and rs2299007 risk alleles create cytosine-phosphate-guanine sites, which are highly methylated and result in lower KIF3A expression, and this methylation is associated with increased transepidermal water loss (TEWL) in risk allele carriers. Kif3a K14 ∆ / ∆ mice have increased TEWL, disrupted junctional proteins, and increased susceptibility to develop AD. Thus, KIF3A is required for skin barrier homeostasis whereby decreased KIF3A skin expression causes disrupted skin barrier function and promotes development of AD. Atopic dermatitis (AD) is the most common chronic inflammatory skin disease, affecting up to 20% of children [1] . Although up to 70% of cases spontaneously remit before adolescence, AD often precedes the development of additional allergic co-morbidities later in life, such as asthma and allergic rhinitis, termed the atopic march [1] . Genetic variation in the cilia structural gene kinesin family number 3A ( KIF3A ) has been associated with AD, asthma, and the atopic march by numerous studies [2] , [3] , [4] , [5] , [6] , [7] , [8] . KIF3A encodes a subunit of the cilia component kinesin-2 and is required for the formation of both motile and nonmotile primary cilia [9] , [10] . Although Kif3a null mice are embryonic lethal [11] , we and others have shown that lung-specific deletion of Kif3a results in barrier dysfunction and unleashes a Th2 allergen response, which contributes to the development of an asthma phenotype [12] , [13] . While KIF3A genetic associations with asthma and AD have been replicated, the mechanism underlying this susceptibility is unknown. Among the KIF3A SNPs associated with asthma and AD, we have found that a third of them create novel cytosine-phosphate-guanine (CpG) sites [7] . CpG regions are prone to modification of the cytosine by the addition of a methyl group to the 5′ position and are known to regulate gene transcription [14] , [15] . In fact, genetic variations have been highly correlated with DNA methylation and CpG sites, linking single nucleotide polymorphisms with epigenetics and gene regulation [16] , [17] . In the present study, we integrate human and mouse studies to dissect the mechanistic basis for the risk conferred by 2 common SNPs in KIF3A for AD. Herein, we show that rs11740584 and rs2299007 AD-risk alleles create new CpG sites, which are highly methylated in individuals carrying one or two copies of the alternate allele. Both SNPs are expression quantitative trait loci (eQTLs) in numerous tissues and allele-specific PCR confirms lower expression from the alternate (risk) allele compared to the reference allele. Methylation levels at these new CpG sites are associated with increased transepidermal water loss (TEWL). These data suggest that KIF3A is required for skin barrier homeostasis and decreased KIF3A expression results in skin barrier dysfunction. In order to investigate causality, we characterize Kif3a K14 ∆/∆ mice. Mice with keratinocyte-selective deletion of Kif3a have increased TEWL and skin thickness, upregulation of the basal marker keratin 5, and dysregulation of adherens and tight junction markers, E-cadherin and claudin-1, respectively. Further, these mice have increased susceptibility to develop features of AD following cutaneous allergen exposure. Thus, rs11740584 and rs2299007 alter the transcriptional regulation of KIF3A , result in decreased KIF3A expression, promote skin barrier dysfunction, and increase susceptibility for AD development. KIF3A is positioned in the 5q31 region, which contains the Th2 cytokine cluster including IL4 and IL13 . As such, the association of KIF3A with allergic outcomes is usually attributed to its proximity to the Th2 gene cluster. Our results highlight the independent role of KIF3A as a key mechanistic pathway for allergic disease pathogenesis and provide insights into the transcriptional regulation of KIF3A . Disease-associated KIF3A SNPs are eQTL KIF3A SNPs rs11740584 and rs2299007 have been associated with asthma and AD [7] , and both are CpG SNPs, such that the alternate or non-reference allele creates a new CpG site (Fig. 1a, b ). Since CpGs undergo epigenetic regulation and impact gene transcription, we utilized Genotype-Tissue Expression Project (GTEx) data [18] , [19] to determine whether rs11740584 and rs2299007 are eQTL. The alternate alleles of rs11740584 and rs2299007 had 14–22% decreased KIF3A expression in sun-exposed and non-sun-exposed skin compared to the reference allele. In the esophagus, the alternate alleles had 26–55% decreased KIF3A expression compared to the reference alleles (Fig. 1c ). Moreover, this effect appeared to be tissue-specific, since the SNPs were strong eQTLs in skin and esophagus, but weaker in the lung. Fig. 1: KIF3A SNPs rs11740584 and rs2299007 create novel CpG sites and are eQTL. a Genomic organization of the human KIF3A and neighboring genes on chromosome 5q31 with the location of SNPs rs11740584 and rs2299007 marked. Magenta bars indicate exons. b Alternate alleles create new CpG sites in both rs11740584 and rs2299007. c Tissue-specific normalized effect size on KIF3A expression data for rs11740584 and rs2299007 were retrieved from the GTEx database, analysis release V7 ( https://www.gtexportal.org ). Each tissue includes biologically independent samples (skin sun exposed n = 605, skin not sun exposed n = 517, esophagus—mucosa n = 497, esophagus—muscularis n = 465 and lung n = 515). The normalized expression values are based on quantile normalization within each tissue and inverse quantile normalization for each gene across samples. The normalized effect size of the eQTL is defined as the effect of the alternate allele relative to the reference allele in the human genome reference GRCh37/hg19. Source data are provided as a Source Data file. Full size image Alternate alleles generate highly methylated CpG sites In order to investigate the mechanistic basis by which rs11740584 and rs2299007 contribute to AD, we recruited individuals carrying 1 or 2 alternate alleles for both SNPs, as well as age- and sex-matched controls who had 2 copies of the reference allele at both SNPs. 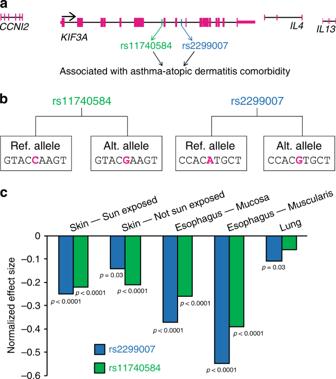Fig. 1:KIF3ASNPs rs11740584 and rs2299007 create novel CpG sites and are eQTL. aGenomic organization of the humanKIF3Aand neighboring genes on chromosome 5q31 with the location of SNPs rs11740584 and rs2299007 marked. Magenta bars indicate exons.bAlternate alleles create new CpG sites in both rs11740584 and rs2299007.cTissue-specific normalized effect size onKIF3Aexpression data for rs11740584 and rs2299007 were retrieved from the GTEx database, analysis release V7 (https://www.gtexportal.org). Each tissue includes biologically independent samples (skin sun exposedn= 605, skin not sun exposedn= 517, esophagus—mucosan= 497, esophagus—muscularisn= 465 and lungn= 515). The normalized expression values are based on quantile normalization within each tissue and inverse quantile normalization for each gene across samples. The normalized effect size of the eQTL is defined as the effect of the alternate allele relative to the reference allele in the human genome reference GRCh37/hg19. Source data are provided as a Source Data file. The study population included 56 individuals between ages 7 and 26 of both white and non-white races (Table 1 ). Since rs11740584 and rs2299007 correlated with decreased expression of KIF3A (Fig. 1c ) and were predicted to create new CpG sites, we hypothesized that the risk alleles for these SNPs may regulate KIF3A expression by altering gene methylation. Given KIF3A association with AD and asthma [7] , [8] , we assessed DNA methylation in skin from adhesive tape strips and in nasal epithelial cells (NEC), from human subjects heterozygous or homozygous for the alternate allele. Individuals with 2 reference alleles for rs11740584 or rs2299007 had either very low or negligible methylation at these loci in both skin and NEC. In contrast, individuals with 1 copy of the alternate allele for rs11740584 had an average of 52 and 43% methylation, while rs2299007 heterozygotes had an average of 16 and 44% methylation in skin and NEC, respectively. Individuals with 2 copies of the alternate allele had a range of 25–78% methylation at the newly-created CpG sites (Fig. 2a–d ). Thus, the alternate alleles for both rs11740584 and rs2299007 created novel CpG sites and these sites were highly methylated in vivo. Our results also indicate that the methylation levels of rs11740584 and rs2299007 are dependent on the number of alternate alleles, since heterozygotes had an average of half of the methylation level observed in homozygotes at each of the novel CpG sites (Fig. 2a–d ). Notably, rs11740584 and rs2299007 genotypes did not result in altered methylation levels at neighboring CpG sites (Supplementary Fig. 1a–c ). These data strongly suggest that these specific SNPs might modify KIF3A expression by changing gene methylation at the newly-created CpG sites and, thus, transcriptional regulation. Table 1 Clinical and demographic characteristics of individuals carrying the reference vs. alternate alleles of KIF3A SNPs rs11740584 and rs2299007. Full size table Fig. 2: rs11740584 and rs2299007 minor allele creates methylated CpG sites and alter KIF3A expression. Skin tape ( a , b ), and nasal epithelial cell ( c , d ), methylation levels at rs11740584 and rs2299007 CpG sites in homozygous and heterozygous alternate allele carriers. A one-way ANOVA was conducted to compare effects of genotype on methylation levels. Each panel includes n = 54 biologically independent samples examined over two independent experiments. Data are presented as mean values ± SD. e Experimental design of allele-specific gene expression illustrating the location of the SNPs, their linkage, and the KIF3A gene. f Fold-change in expression in nasal epithelial and primary keratinocyte cells are provided relative to the C allele. Data are presented as mean values ± SD of three individuals in technical quadruplicates examined over two independent experiments per tissue type. Linear mixed models were performed to access the expression difference between risk allele and reference allele. P values of two-sided testing were reported for all the tests. NEC = nasal epithelial cells. Source data are provided as a Source Data file. Full size image rs11740584 alternate allele decreases KIF3A expression We next utilized allele-specific qPCR to determine whether rs11740584 directly impacts KIF3A expression. Since rs11740584 and rs2299007 are intronic and, therefore, not transcribed in messenger RNA, we identified a genetic variant (rs17690965) located within a KIF3A exon, which is in strong LD with rs11740584 ( r 2 = 0.96) (Fig. 2e ). With allelic qPCR, we observed a 17% decrease in KIF3A expression for the alternate allele G relative to the reference allele C in NEC derived from three heterozygote individuals ( p = 0.0064, linear mixed models) (Fig. 2f ). We also assessed allele-specific expression in primary human keratinocytes derived from 3 donors heterozygous for rs11740584 and found 19% less expression from the risk allele ( p = 0.0019, linear mixed models) (Fig. 2f ). Thus, the rs11740584 alternate allele results in lower KIF3A gene expression compared to the reference allele in primary keratinocytes and upper respiratory NEC. These data are consistent with the GTEx data where the alternate alleles of rs11740584 and rs2299007 were associated with 14–22% decreased expression (Fig. 1c ). No coding genetic variant in strong LD was identified for rs2299007. In silico analysis of rs11740584 and rs2299007 Since rs11740584 and rs2299007 were associated with increased CpG methylation and decreased expression, we conducted an in silico analysis in order to identify particular transcription factors (TFs) whose binding sites might be altered by the rs11740584 and rs2299007 genetic variants using the CisBP web [20] and the findings are summarized in Supplementary Table 1 . Strikingly, the non-reference (G) allele creates a perfect (consensus) E-box binding site (CACATG changed to CACGTG). Further, ChIP-seq peaks for the MYC E-box binding protein are present in BJ cells (foreskin fibroblast cell line), indicating that MYC is capable of binding this locus in a cellular context [21] . Basic helix-loop-helix (bHLH) family TFs such as MYC can bind the CACGTG E-box when the CpG is methylated [22] . Neither SNP has histone marks in relevant (skin or lung) cell types. The non-reference (risk) allele for rs11740584 creates a binding site for the transcription factor ZSCAN26 (Supplementary Table 1 ). Methylation levels are associated with increased TEWL We observed that presence of KIF3A SNPs rs11740584 and rs2299007 created highly methylated CpG sites and resulted in the downregulation of KIF3A expression by about 17–19%. Since these SNPs were strongly associated with AD, we hypothesized that these epigenetic changes in KIF3A might be correlated with disrupted skin barrier function in individuals carrying the alternate alleles. To address this, we directly compared skin TEWL and rs11740584 and rs2299007 methylation levels. 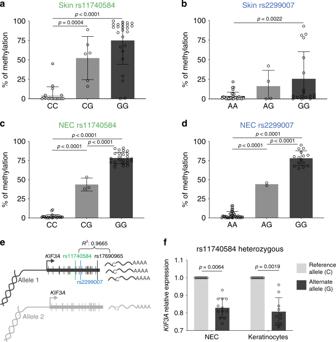Fig. 2: rs11740584 and rs2299007 minor allele creates methylated CpG sites and alterKIF3Aexpression. Skin tape (a,b), and nasal epithelial cell (c,d), methylation levels at rs11740584 and rs2299007 CpG sites in homozygous and heterozygous alternate allele carriers. A one-way ANOVA was conducted to compare effects of genotype on methylation levels. Each panel includesn= 54 biologically independent samples examined over two independent experiments. Data are presented as mean values ± SD.eExperimental design of allele-specific gene expression illustrating the location of the SNPs, their linkage, and theKIF3Agene.fFold-change in expression in nasal epithelial and primary keratinocyte cells are provided relative to the C allele. Data are presented as mean values ± SD of three individuals in technical quadruplicates examined over two independent experiments per tissue type. Linear mixed models were performed to access the expression difference between risk allele and reference allele.Pvalues of two-sided testing were reported for all the tests. NEC = nasal epithelial cells. Source data are provided as a Source Data file. Methylation levels in the skin of the novel CpG sites created by rs11740584 and rs2299007 were significantly associated with skin barrier dysfunction as assessed by TEWL values ( p = 0.01 and 0.0004, respectively, generalized linear models) in human carriers of the risk alleles (Table 2 ). Table 2 KIF3A SNPs rs11740584 and rs2299007 methylation levels are associated with higher transepidermal water loss (TEWL). Full size table Kif3a is required for skin barrier homeostasis and function In order to directly prove that reduced Kif3a expression causes skin barrier dysfunction, we generated Kif3a K14 ∆/∆ mice with epidermis-specific deletion of Kif3a . Kif3a K14 ∆/∆ mice had higher TEWL compared to Kif3a +/+ control mice ( p < 0.0001, one-way ANOVA) (Fig. 3a ) demonstrating skin barrier disruption. Notably, intermediate TEWL measurements were observed in Kif3a K14 ∆/+ mice and were significantly elevated compared to control mice, supporting a gene dosage effect ( p < 0.01, one-way ANOVA). In fact, we found that skin barrier integrity, assessed by TEWL, was inversely correlated to skin Kif3a mRNA levels ( p < 0.0001, one-way ANOVA) (Fig. 3b, c ). Histological examination of skin sections showed intermittent regions of increased thickness in Kif3a K14 ∆/∆ adult mice relative to Kif3a +/+ littermates. The typically very thin epidermis in haired areas was increased from the normal 2–3 cell layers to up to 6 cells in thickness. Parakeratosis, hyperkeratosis, and hypergranulosis were focally present in Kif3a K14 ∆/∆ mice with these findings being rare in Kif3a +/+ mice (Fig. 3d, e ). Epithelial hyperplasia was uniformly present in Kif3a K14 ∆/∆ mice analyzed at 3 weeks, 5 weeks, and 8 weeks of age and was not seen in age matched Kif3a +/+ mice (Supplementary Fig. 2a, b ). Consistent with what we observed with TEWL, the Kif3a K14 ∆/+ mice had intermediary epidermal thickness between the Kif3a K14 ∆/∆ and Kif3a +/+ mice (Fig. 3e ). To address whether epidermal thickness was a result of increased cell proliferation, we carried out immunostaining with Ki67. In 3 week old mice, there was a significant increase in the percentage of Ki67 positive cells in the interfollicular epidermis of Kif3a K14 ∆/∆ compared to Kif3a +/+ animals (Fig. 3f ; p = 0,0025, t test). This difference was no longer evident at 8 weeks of age (Fig. 3f ) suggesting that the increased epidermal thickness observed in 8-week old animals might be a result of the earlier cell proliferation. Fig. 3: Kif3a K14 ∆/∆ mice develop disrupted skin barrier. a Trans-epidermal water loss (TEWL) was measured in Kif3a +/+ , Kif3a ∆/+ and Kif3a K14 ∆/∆ mice, age 6–10 weeks ( n = 284 biologically independent animals examined over three independent experiments). b RNA isolated from Kif3a +/+ , Kif3a ∆/+ , and Kif3a K14 ∆/∆ epidermis was assessed for mRNA levels of Kif3a . Values are expressed as fold change over Kif3a +/+ and relative to Hprt ( n = 29 biologically independent animals examined over three independent experiments). A one-way ANOVA was conducted to compare the effects of genotype on TEWL and gene expression. c Linear correlation between TEWL and Kif3a expression in Kif3a +/+ , Kif3a ∆/+ , and Kif3a K14 ∆/∆ mice ( n = 30 biologically independent animals examined over three independent experiments). Spearman correlation was conducted to compare TEWL and Kif3a expression. d Representative H&E staining and e epidermal thickness of Kif3a +/+ , Kif3a ∆/+ , and Kif3a K14 ∆/∆ mice at 8 weeks of age ( n = 28 biologically independent animals examined over three independent experiments). Scale bar: 100 μm. A one-way ANOVA was conducted to compare effects of genotype on epidermal thickness. f Ki67 quantification on epidermis sections from 3 and 8 week old Kif3a +/+ and Kif3a K14 ∆/∆ mice ( n = 11 and n = 17 biologically independent animals examined over two independent experiments, respectively). T test was conducted to compare effects of genotype on Ki67 expression. P values of two-sided testing were reported for all the tests. Data in all panels are presented as mean values ± SD. Source data are provided as a Source Data file. Full size image Kif3a -deficient skin has abnormal epidermal cell adhesion Given the disrupted skin barrier observed in the Kif3a K14 ∆/∆ mice, we next performed transcriptome analyses of the epidermis to gain insights into the observed phenotype in the mice. RNA-seq was performed on 8 week old Kif3a +/+ and Kif3a K14 ∆/∆ epidermis. Analysis of differential gene expression revealed 394 downregulated and 408 upregulated genes in the absence of Kif3a (Supplementary Fig. 3a–c ). Among the top functional terms represented in the downregulated genes were regulation of defense mechanisms, cell adhesion molecule binding, and response to wounding. Meanwhile, the top functional terms among the upregulated genes were growth factor binding and basolateral membrane (Supplementary Fig. 3d ). Epidermal expression of Irf4 , Wnt7a , and Kng2 were downregulated, confirming the downregulation of defense and wound response genes in the absence of Kif3a . Meanwhile markers for response to sterol and growth factor binding Inhba , Ntrk4 , and Igfals were upregulated in the absence of Kif3a (Supplementary Fig. 3e ). Collectively, the RNA-seq data indicate skin morphological changes with increased expression of genes expressed in the basolateral membrane and decreased expression of cell adhesion genes in the absence of Kif3a , thus we assessed the distribution of basal cell marker keratin 5, as well as adherens junction and tight junction markers E-cadherin and claudin1 in Kif3a +/+ and Kif3a K14 ∆/∆ mice. Confocal imaging of skin sections stained for keratin 5 revealed an expansion of the basal layer from 1 to 2 cells found in Kif3a +/+ animals, to 5–6 cells in Kif3a K14 ∆/∆ (Fig. 4 ). Expression of E-cadherin and claudin1 was drastically diminished in the basal cells of Kif3a K14 ∆/∆ epidermis compared to the even distribution in wild types (Fig. 4 ). Overall, these data strongly support a role for Kif3a in skin homeostasis, whereby loss of Kif3a results in over proliferation of the basal cell layer and altered localization of adherens and tight junction proteins that likely contribute to the observed higher TEWL at baseline. Fig. 4: Kif3a K14∆/∆ mice have disrupted adherens junction and tight junction markers. Epidermis sections from 8 to 10 week old Kif3a +/+ and Kif3a K14 ∆/∆ mice were stained for basal cell marker keratin 5, adherens junction E-cadherin, and tight junction claudin-1, and imaged by confocal microscopy. DAPI was used as nuclei marker. Data shown here is maximum intensity projection. ( n = 15 biologically independent animals examined over two independent experiments). Scale bar: 100 μm. Full size image Kif3a K14 ∆/∆ mice are prone to develop an AD-like phenotype Since KIF3A has been identified as a susceptibility gene for AD [2] , [3] , [4] , [5] , [6] , [7] , [8] and our data revealed that its deficiency causes skin barrier dysfunction, we reasoned that Kif3a K14 ∆/∆ mice may have increased susceptibility to develop AD. Kif3a K14 ∆/∆ mice skin appeared normal without lesions or erythema by H&E staining (Fig. 3d ) and no baseline inflammation was observed in the skin by IL-4 and IL-13 qPCR, and CD3 staining (Supplementary Fig. 4 ). Therefore, we used a cutaneous allergen exposure of Aspergillus fumigatus , to model AD. In this model, cutaneous applications of Asp. fumigatus result in increased TEWL, allergic sensitization, skin erythema, skin thickness, and Th2 responses, all landmarks of AD, without the need for prior mechanical tape stripping or skin perturbation with shaving creams needed in other models [23] , [24] , [25] . Upon one week of skin patching, Kif3a K14 ∆/∆ developed increased TEWL after cutaneous exposure to Aspergillus fumigatus allergen compared to Kif3a +/+ mice (Fig. 5a ). Epidermal thickness was also significantly increased in Kif3a K14 ∆/∆ mice compared to Kif3a +/+ mice upon cutaneous allergen exposure (Fig. 5b, c ). Thus, Kif3a K14 ∆/∆ mice have a disrupted skin barrier and, while they do not have AD at baseline, they are more susceptible to develop AD-like features upon cutaneous allergen exposure than their wild type counterparts. Fig. 5: Kif3a K14 ∆/∆ mice are more prone to develop AD-like phenotype following cutaneous allergen exposure. a TEWL measurement at 8 weeks of age in Kif3a +/+ and Kif3a K14 ∆/∆ mice sensitized with saline control or Aspergillus fumigatus ( n = 78 biologically independent animals examined over three independent experiments). b Epidermal thickness and c representative H&E staining of skin samples of Kif3a +/+ and Kif3a K14 ∆/∆ mice sensitized with Aspergillus fumigatus ( n = 31 biologically independent animals examined over three independent experiments). Scale bars, 50 μm. A one-way ANOVA was conducted to compare effects of genotype and/or treatment on TEWL and epidermal thickness. P values of two-sided testing were reported for all the tests. Data in all panels are presented as mean values ± SD. Source data are provided as a Source Data file. Full size image Our data provide a mechanistic basis for the AD disease susceptibility conferred by KIF3A SNPs rs11740584 and rs2299007 whereby the alternate alleles generate new CpG sites resulting in increased methylation and decreased expression of KIF3A . Skin methylation of the novel CpG sites created by rs11740584 and rs2299007 was associated with increased TEWL in individuals carrying the risk alleles. To prove causality, we characterized mice with tissue-specific deficiency of Kif3a in keratinocytes. Kif3a K14 ∆/∆ mice had skin barrier dysfunction at baseline as evidenced by increased TEWL and epidermal thickness and disrupted basal cell, adherens and tight junctional protein expression. Finally, the skin barrier dysfunction observed in Kif3a K14 ∆/∆ mice is disease relevant as these mice had increased susceptibility to develop AD features upon cutaneous allergen exposure. Thus, KIF3A deficiency causes skin barrier dysfunction and contributes to AD susceptibility (Fig. 6 ). Fig. 6: Mechanistic underpinnings of the contribution of KIF3A SNPs rs11740584 and rs2299007 to skin barrier dysfunction. Allergic disease-associated KIF3A SNPs create new CpG sites, which are highly methylated in individuals carrying the alternate allele leading to decreased KIF3A expression. Decreased KIF3A results in increased TEWL due to defective cell-cell adhesion, and increased susceptibility to the development of AD. ALRG = allergen. Full size image Previous work by our group and others has shown that KIF3A is a susceptibility gene for AD and asthma [2] , [3] , [4] , [5] , [6] , [7] , [8] , however, until now, the mechanistic basis for this association has been unclear. KIF3A rs11740584 and rs2299007 alternate alleles are predicted to create new CpG sites. Although CpG regions are susceptible to DNA methylation, they do not necessarily receive the methyl group [14] , [15] , [26] , thus the generation of a CpG does not mean that they are actually methylated in vivo. However, we found that alternate allele carriers for rs11740584 and rs2299007 had 25–78% methylation at each of these sites (vs. 2–5% in reference allele carriers). The high methylation level at these SNP loci in human alternate allele carriers suggests that these SNPs are important in the transcriptional regulation of KIF3A . Indeed, both rs11740584 and rs2299007 are eQTLs for KIF3A in different tissues of interest and allele-specific PCR revealed that rs11740584 alternate allele results in up to 19% less KIF3A expression. The non-reference (G) risk allele for rs2299007 creates a CACGTG E-box. Basic helix-loop-helix (bHLH) family TFs, such as MYC can bind the CACGTG E-box when the CpG is methylated [22] . So, the prediction would be that the rs2299007 non-reference risk allele creates a binding site for MYC, and MYC binds this site more strongly. Indeed, rs2299007 is located inside of a MYC ChIP-seq peak in fibroblasts [21] . Collectively, these findings add a layer to what is currently known regarding KIF3A transcriptional regulation and further highlight the relevance of our findings. Chromatin modifications, and RNA polymerase II loading have all been shown to be modified by SNPs [27] , [28] , and could be the link between these variants and transcriptional regulation. Our data demonstrate that the new sites are methylated in alternate allele carriers, while they are not methylated in reference allele carriers. Thus, KIF3A rs11740584 and rs2299007 genotypes predict the methylation status at the SNP site and support a role in KIF3A gene expression regulation. Although we showed strong evidence for this correlation, we did not directly test that methylation is associated with expression independent of genotype. It remains to be elucidated how KIF3A rs11740584 and rs2299007 CpG methylation alters KIF3A expression and what the transcriptional regulatory events are that mediate this process. While our data demonstrate that KIF3A can contribute to AD development, it is important to note that KIF3A or any single factor is highly unlikely to be solely responsible for AD development. KIF3A is a component of the primary cilia, which are sensory structures that transduce extracellular signals to the cell interior [9] , [10] , and in Kif3a absence, this microtubule-based structure is not formed properly [29] . Because Kif3a is important for the primary cilia structure, signaling pathways like Shh, Wnt, and Notch, that rely on this sensory organ [30] , [31] , [32] , might be related to the phenotype described in the present study. Indeed, mice deficient in Notch signaling develop dry skin, barrier abnormalities, and increased TEWL just like reported in the current study [33] , [34] . Therefore, the role of Kif3a in the primary cilia may be to connect different signaling pathways suggesting a complex and intricate regulatory network, that remains to be investigated. Since KIF3A methylation at the newly generated rs11740584 and rs2299007 CpG sites was highly correlated with skin barrier dysfunction, specifically increased TEWL, KIF3A genotype and/or methylation at these sites may be clinically useful biomarkers of AD development in pregnancy or early life. This is highly relevant because AD is a significant risk factor for food allergy development, as it has been widely described and systematically reviewed recently [35] . Food allergy prevalence is on the rise, and the development and implementation of strategies for food allergy prevention will require tools to accurately predict which children will develop AD. Indeed, the cytokine gene cluster on chromosome 5q31.1, where KIF3A is located, has been associated with food allergies in a GWAS (genome-wide association study) study [36] . Our findings provide insights into the transcriptional regulation of KIF3A . The linkage of chromosomal region 5q31 and the linkage of this locus to allergic disease has been largely attributed to the Th2 cytokine gene cluster [8] , [37] , [38] . Our results in mice highlight the independent role of KIF3A as a key mechanistic pathway for allergic disease susceptibility and provide insights into the transcriptional regulation of KIF3A as wells as a potential new target for the prevention and treatment of AD. Subjects The GCPCR- KIF3A cohort included a total of 56 participants, 45 children aged 7–17 years old and 11 adults aged 18–26 years old from the greater Cincinnati, Ohio metro area who were initially enrolled in either the Greater Cincinnati Pediatric Clinic Repository (GCPCR), Genomic Control Cohort (GCC), Cincinnati Childhood Allergy and Air Pollution Study (CCAAPS), or the Cincinnati Center for Eosinophilic Disorders (CCED) cohorts, which have been extensively described previously [5] , [39] , [40] . Based on genotyping information available from these cohorts, we recruited individuals based on genotype for KIF3A SNPs rs11740584 and/or rs2299007. Cases carried at least alternative allele for one of these SNPs, controls did not carry alternatives alleles for either SNP. The cases and controls were matched on age, sex, and allergic disease status. The subjects or their legally authorized representatives (LARs) completed our validated New Visit Questionnaire (NVQ) [39] , which collects information regarding AD, allergic rhinitis, food allergy, asthma and allergy symptoms, medical history, family history of allergic disease, medications, diet, home characteristics, and environmental exposures. Subjects also completed our Demographic Data Questionnaire (DDQ) [39] , which captures age, sex, race, and ethnicity of the participant and participant’s parents and socioeconomic status indicators. Study approval GCPCR- KIF3A subjects, or their LAR, provided informed consent or parental permission/assent, respectively, prior to inclusion in the study. The study was approved by the Cincinnati Children’s Hospital Medical Center Institutional Review Board under protocol number 2010-0438. Primary human keratinocytes were isolated from de-identified human discard skin isolates from plastic surgeries at University of Cincinnati, Cincinnati Children’s Hospital Medical Center and Shriners Hospital. The study was approved by the University of Cincinnati Institutional Review Board under protocol number 2013-4582 and determined as “non-human subjects research” by the University of Cincinnati Institutional Review Board. Mice were maintained and handled according to the Guide for the Care and Use of Laboratory Animals (Institute of Laboratory Animal Resources, National Research Council). All animal procedures were approved by the Institutional Animal Care and Use Committee (Cincinnati Children’s Hospital Medical Center). Human transepidermal water loss (TEWL) Water loss was measured using the SkinLab Combo and based on Nilsson’s Vapor Pressure Gradient method. Measurements were made according to published guidelines [41] . The temperature and the relative humidity of the rooms where measurements were made varied between approximately 20 and 27 °C and 10% and 60% relative humidity. Median values of temperature and relative humidity did not differ significantly either between cases and controls (Supplementary Table 2 , Wilcoxon test). Subjects had not used any topical ointment, cream, lotion or moisturizer for at least 12 h prior to the measurement, by their report. TEWL measurements were taken after an acclimatization period of at least 15 min. Measurements were recorded as g/m 2 /h after the rate of TEWL had stabilized, approximately after 60 s and when the standard deviation became 0.2 or less. The volar forearm sites were assessed for TEWL. The same coordinator measured TEWL on all study subjects. TEWL measurements were corrected for day-to-day variation by normalization to one control subject whose TEWL was measured within 30 min of every subject. Human skin sampling and DNA extraction Skin cells were collected with adhesive SmartSolve Strips pre-cut into eleven 1 × 1 inch strips. The tape strips were placed adhesive side down on (volar forearm) and massaged for 20 s. The location of the first tape was outlined on the skin and subsequent tapes were applied at the same location. Tapes are collected in BL + TG buffer (4 M guanidine thiocyanate, 0.01 M Tris (pH7.5) and 2% 1-thioglycerol), flash frozen and stored at −80 °C. Genomic DNA was isolated from tape strips using the Promega Wizard DNA isolation kit (Madison, WI). Human nasal epithelial cells collection and DNA/RNA extractions NEC sampling was performed by using a CytoSoft Brush (Medical Packaging Corp) and the sample was immediately placed on ice in 10%ß-ME in RLT buffer (Qiagen AllPrep DNA/RNA Micro Kit). Within 30 min of collection, the sample was flash frozen with dry ice and stored at −80 °C. DNA and RNA were extracted using the AllPrep DNA/RNA Micro Kit (Qiagen). Bisulfite pyrosequencing For DNAm measurement, 300 ng genomic DNA was subjected to sodium bisulfite treatment and purified using the EZ DNA methylation-Gold Kit (Zymo Research) according to the manufacturer’s specifications. 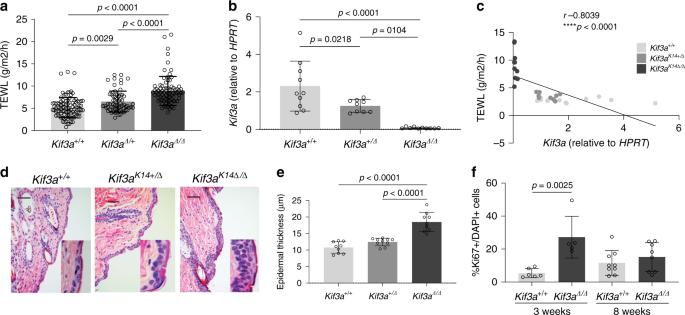Fig. 3:Kif3aK14∆/∆mice develop disrupted skin barrier. aTrans-epidermal water loss (TEWL) was measured inKif3a+/+,Kif3a∆/+andKif3aK14∆/∆mice, age 6–10 weeks (n= 284 biologically independent animals examined over three independent experiments).bRNA isolated fromKif3a+/+,Kif3a∆/+, andKif3aK14∆/∆epidermis was assessed for mRNA levels ofKif3a. Values are expressed as fold change overKif3a+/+and relative toHprt(n= 29 biologically independent animals examined over three independent experiments). A one-way ANOVA was conducted to compare the effects of genotype on TEWL and gene expression.cLinear correlation between TEWL andKif3aexpression inKif3a+/+,Kif3a∆/+, andKif3aK14∆/∆mice (n= 30 biologically independent animals examined over three independent experiments). Spearman correlation was conducted to compare TEWL andKif3aexpression.dRepresentative H&E staining andeepidermal thickness ofKif3a+/+,Kif3a∆/+, andKif3aK14∆/∆mice at 8 weeks of age (n= 28 biologically independent animals examined over three independent experiments). Scale bar: 100 μm. A one-way ANOVA was conducted to compare effects of genotype on epidermal thickness.fKi67 quantification on epidermis sections from 3 and 8 week oldKif3a+/+andKif3aK14∆/∆mice (n= 11 andn= 17 biologically independent animals examined over two independent experiments, respectively).Ttest was conducted to compare effects of genotype on Ki67 expression.Pvalues of two-sided testing were reported for all the tests. Data in all panels are presented as mean values ± SD. Source data are provided as a Source Data file. Bisulfite DNA was amplified with ZymoTaq PreMix (Zymo Research) with the primer sets listed in the Supplementary Table 3 . Pyrosequencing was carried out using Pyro Gold reagents with a PyroMark vacuum prep workstation and a PyroMark Q96 MD instrument (Qiagen) following the manufacturer’s instructions. The generated pyrograms were automatically analyzed using Pyro Q-CpG methylation analysis software (Qiagen, Version 1.0.11). 100% methylation control (SssI-treated human genomic DNA) and 0% methylation control (human genomic DNA amplified by GenomePlex® Complete WGA kit (Sigma) were used in validating all assays. Primary human keratinocytes strains Primary human keratinocytes were isolated from de-identified human skin discarded from breast reductions performed in healthy females. Cells were isolated from human epidermis, and were confirmed to be keratinocytes based on morphology and growth characteristics in selective culture media. Allelic qPCR The SNPs rs11740584 and rs2299007 are intronic and, therefore, not transcribed in messenger RNA, so we identified a genetic variant (rs17690965) in strong LD with rs11740584 ( r 2 = 0.96) located within a KIF3A exon. No genetic variant in strong LD was found for rs2299007 to perform this analysis. NEC and primary human keratinocytes mRNA was used to perform reverse transcriptase reaction with the SuperScript IV VILO Master Mix (Invitrogen). Allele-specific qPCR was performed with Taqman genotyping primers (ThermoFisher) for rs17690965 on keratinocytes and NEC cDNA and genomic DNA of three heterozygote individuals each who carried one alternate and one reference allele. Primer/probe is listed in Supplementary Table 3 . Fold change of expression was calculated with 2 −ΔΔCT values, where cDNA was normalized to gDNA. KIF3A associated SNPs in silico transcription factor binding site analysis We sought to identify particular transcription factors (TFs) whose binding sites might be altered by the rs11740584 and rs2299007 genetic variants using the CisBP web [20] . Generation of Kif3a K14 ∆/∆ mice with targeted deletion of Kif3a in the skin Skin-specific conditional Kif3a knockout mice were generated by breeding K14-Cre;R26R-eYFPflox-stop-flox mice [42] to Kif3a flox/flox mice [43] . In the presence of K14-driven Cre-recombinase, flox-flanked exon 2 of the Kif3a gene was deleted in epidermal cells introducing a frameshift in the coding region resulting in premature termination of Kif3a translation. Kif3a K14 ∆/∆ mice were maintained on an alternating 12-h light cycle with food and water ad libitum, the temperature was kept between 70 and 74 F and humidity between 30 and 70%, and otherwise maintained and handled according to the Guide for the Care and Use of Laboratory Animals (Institute of Laboratory Animal Resources, National Research Council). Mice measurement of TEWL TEWL was measured by using DermaLab’s instrument (Cortex Technology). The temperature and relative humidity in the rooms are held constant. Mice were shaved one day before the measurement. 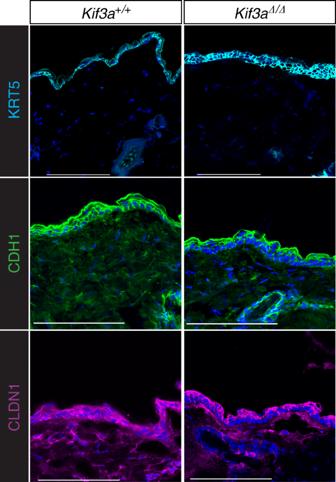Fig. 4:Kif3aK14∆/∆mice have disrupted adherens junction and tight junction markers. Epidermis sections from 8 to 10 week oldKif3a+/+andKif3aK14∆/∆mice were stained for basal cell marker keratin 5, adherens junction E-cadherin, and tight junction claudin-1, and imaged by confocal microscopy. DAPI was used as nuclei marker. Data shown here is maximum intensity projection. (n= 15 biologically independent animals examined over two independent experiments). Scale bar: 100 μm. TEWL was assessed by placing the probe against the shaved skin surface in the center of the back area. Measurements were recorded in g/m 2 /h. TEWL numbers were read twice and the average was recorded. Mice skin RNA isolation and quantitative real time PCR Total RNA was isolated from homogenized mouse skin using RNeasy Microarray Tissue Mini Kit (Qiagen) according to manufactures’ instructions. Skin RNA was used to perform reverse transcriptase reaction with the SuperScript IV VILO Master Mix (Invitrogen). Taqman primer/probes for HPRT, Kif3a, IL4, IL13, Irf4, Wnt7a, Kng2, Inhba, Ntkr2 , and Igfals are listed in Supplementary Table 3 . Primers/probes were used following the manufacturer’s instructions. HPRT was used as a housekeeping gene to normalize the expression of all genes. Mice epidermis RNA isolation Epidermis from 8 week old Kif3a +/+ and Kif3a K14 ∆/∆ animals were isolated with the use of dispase. Total RNA was isolated from homogenized skin using RNeasy Microarray Tissue Mini Kit (Qiagen) according to the manufactures’ instructions. RNA-seq Skin mRNA from six Kif3a +/+ and six Kif3a K14 ∆/∆ were submitted to RNA-seq at the Genomics, Epigenomics and Sequencing Core at the University of Cincinnati. The RNA quality was determined by Bioanalyzer (Agilent, Santa Clara, CA). NEBNext Poly(A) mRNA Magnetic Isolation Module (New England BioLabs, Ipswich, MA) was used to isolate polyA RNA. Library was prepared with NEBNext Ultra II Directional RNA Library Prep Kit (New England BioLabs) and sequenced using HiSeq 1000 sequencer (Illumina, San Diego, CA). Each sample had around 25 million single reads at 51 bp long. Quality trimmed reads were mapped to the mm10 genome, quantified using RSEM and mapped with Bowtie 2 using default thresholds [44] . Differential gene expression analysis was carried out with RUVSeq [45] with log2 fold change (FC) ≥ 1 or ≤ −1, P < 0.05 and false discovery rate (FDR) ≤ 5%. 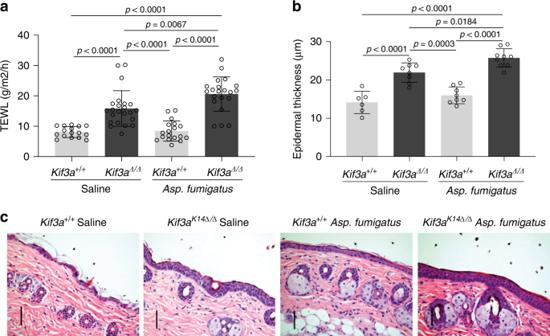Fig. 5:Kif3aK14∆/∆mice are more prone to develop AD-like phenotype following cutaneous allergen exposure. aTEWL measurement at 8 weeks of age inKif3a+/+andKif3aK14∆/∆mice sensitized with saline control orAspergillus fumigatus(n= 78 biologically independent animals examined over three independent experiments).bEpidermal thickness andcrepresentative H&E staining of skin samples ofKif3a+/+andKif3aK14∆/∆mice sensitized withAspergillus fumigatus(n= 31 biologically independent animals examined over three independent experiments). Scale bars, 50 μm. A one-way ANOVA was conducted to compare effects of genotype and/or treatment on TEWL and epidermal thickness.Pvalues of two-sided testing were reported for all the tests. Data in all panels are presented as mean values ± SD. Source data are provided as a Source Data file. 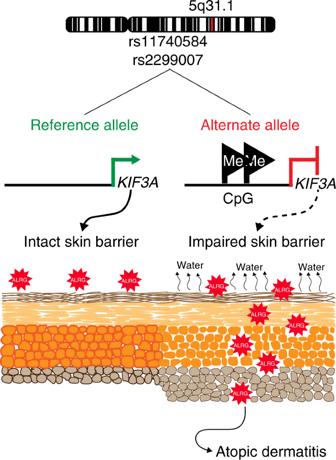Fig. 6: Mechanistic underpinnings of the contribution ofKIF3ASNPs rs11740584 and rs2299007 to skin barrier dysfunction. Allergic disease-associatedKIF3ASNPs create new CpG sites, which are highly methylated in individuals carrying the alternate allele leading to decreasedKIF3Aexpression. DecreasedKIF3Aresults in increased TEWL due to defective cell-cell adhesion, and increased susceptibility to the development of AD. ALRG = allergen. Volcano Plots were generated using CSBB’s InteractiveScatterPlot module. GO term enrichment analyses were performed using WebGestalt [46] . Heatmaps were generated using GeneE from Broad Institute ( https://software.broadinstitute.org/GENE-E/index.html ). Mice skin histology Skin tissues were fixed in 10% formalin immediately after mice were euthanized. Paraffin-embedded tissues were cut into 5 µm sections and stained with H&E for histology and to assess skin thickness. Epidermal thickness was quantified using morphometric software (Metamorph) and an average of 10 random fields (×200) were measured for each sample. T cells were assessed by immunohistochemistry using anti-CD3 (Biolegend). Positive cells were quantified under microscope for 10 to 15 random fields (×200) and results were expressed as cells per field. Immunostaining and imaging experiments Immunostaining experiments were carried out on 7 micron frozen sections of mice epidermis. Air-dried frozen sections were post fixed in 4% paraformalydehyde. Sections were incubated with following primary antibodies: Keratin 5 (905501, Rabbit polyclonal, Biolegend), E-cadherin (180223, Mouse monoclonal IgG1kappa, Life technologies), Claudin 1 (37-4900, Mouse IgG1, Thermofisher Scientific), Ki67 (ab15580, Rabbit polyclonal, Abcam). Primary antibodies were used at 1:200 dilution in 4% NGS block overnight. Sections were incubated with the following secondaries: Alexafluor 488 anti-rabbit (A-11008, Thermofisher Scientific), Alexafluor 488 (A-11029, Thermofisher Scientific), Alexafluor 594 anti-mouse (A-11032, Thermofhisher scientific) and nuclear stain DAPI at 1:200. Confocal imaging was performed using the Nikon TI-E Inverted microscope at the Cincinnati Children’s Confocal Imaging Core. Images were analyzed using the Nikon Imaging Software Elements (Version 4.4) and ImageJ (Version 1.52) was used to quantify immunostaining images as appropriate. Mice epicutaneous exposure to aspergillus fumigatus Mice were shaved on their backs a day before the allergen exposure. Sterile 2 × 2 cm gauzes moistened with 200 μg Aspergillus fumigatus spore extract (Greer Laboratories) in phosphate-buffered saline was applied to the shaved area. The patch was secured with TegaDerm and a bandaid was placed around the mouse waist. After 6 days the patch was removed, and 24 h later TEWL was measured over the exposed area. Statistical analysis Descriptive statistics were used to characterize the study population. Frequencies (percentage) were reported for categorical variables while geometric means and confidence intervals (CI) were reported for continuous variables as data were log transformed to improve distributional characteristics. Generalized Linear Models with gaussian distribution and log link function were fitted to examine the SNP methylation association with TEWL. The associations between KIF3A SNPs genotypes and their methylation were tested using one-way ANOVA. To compare KIF3A allelic expression differences, we first standardized the expression data for each person to ensure that the expression data were in the same scale and comparable using the scale function in R. Linear mixed models were performed to access the expression difference between risk allele and reference allele, assuming a positive-definite symmetrical correlation matrix for the two conditions. “Person” was included as a random effect in the (linear mixed) model to account for the correlations among the replicates for each person. Replicate values from 2 different individuals that exceeded a coefficient of variation of 10 were removed. Linear regression was used for the mice analysis to examine Kif3a association with TEWL. A one-way ANOVA was conducted to compare effects of genotype on TEWL, gene expression and epidermal thickness (8 week old). T test was conducted to compare effects of genotype on Ki67 expression and epidermal thickness (3 and 5 week old). A nominal p value threshold ( p < 0.05) was applied for significance. P values of two-sided testing were reported for all the tests. All analyses were performed in R software, version 3.3.2 ( https://www.r-project.org ). Reporting summary Further information on research design is available in the Nature Research Reporting Summary linked to this article.